The C-terminal helical bundle of the tetrameric prokaryotic sodium channel accelerates the inactivation rate Most tetrameric channels have cytosolic domains to regulate their functions, including channel inactivation. Here we show that the cytosolic C-terminal region of NavSulP, a prokaryotic voltage-gated sodium channel cloned from Sulfitobacter pontiacus , accelerates channel inactivation. The crystal structure of the C-terminal region of NavSulP grafted into the C-terminus of a NaK channel revealed that the NavSulP C-terminal region forms a four-helix bundle. Point mutations of the residues involved in the intersubunit interactions of the four-helix bundle destabilized the tetramer of the channel and reduced the inactivation rate. The four-helix bundle was directly connected to the inner helix of the pore domain, and a mutation increasing the rigidity of the inner helix also reduced the inactivation rate. These findings suggest that the NavSulP four-helix bundle has important roles not only in stabilizing the tetramer, but also in accelerating the inactivation rate, through promotion of the conformational change of the inner helix. Voltage-gated sodium channels have essential roles in many important physiological processes, such as electric signalling, muscle contraction, and pain sensation [1] . Their subtypes also show various channel properties, such as voltage dependency and the kinetics of activation and inactivation, characterizing their unique function. Therefore, mutations that impair channel activity can cause serious channelopathies [2] , [3] . Prokaryotic voltage-gated sodium channels (NavBacs) are simple tetrameric sodium channels comprising monomers shorter than 300 amino acids [4] , [5] , [6] , [7] . Each subunit contains 6 transmembrane α-helices (S1–S6). Helices S5 and S6 form the pore domain in the centre of the tetrameric channel, and helices S1–S4 form voltage sensors that surround the pore domain and detect the membrane potential. NavBacs are widespread in various bacteria and small changes in their primary sequences alter their channel properties depending on the host bacteria environment [4] , [5] , [6] , [7] . Their various channel properties and structural simplicity make NavBacs useful for analysing the basic molecular mechanisms of voltage-gated sodium channels. Recently, the crystal structure of NavAb, cloned from Arcobacter butzleri , was determined by X-ray crystallography [8] . The crystal structure provided the first insight into the characteristic features of Nav channels, such as the additional helix (P2-helix) in the extracellular vestibule of the pore domain and fenestrations on the sides of the pore module. The structure of the cytosolic carboxy-terminal region of NavAb, however, was unclear [8] . Almost all known ion channels contain cytoplasmic domains that have essential roles in forming tetramers [9] , channel gating [10] , [11] , and regulating channel function [12] , [13] . On the basis of electrophysiological analyses, as well as determination of the crystal structure of the C-terminal region of NavSulP grafted into the C-terminus of the NaK channel, we provide evidence that the cytosolic C-terminal region of NavSulP, which is cloned from Sulfitobacter pontiacus , accelerates the channel inactivation rate. The C-terminal region of NavSulP stabilized the tetrameric channel by forming a four-helix bundle (4HB). Moreover, the NavSulP 4HB formation had a unique role to accelerate the inactivation rate through a conformational change of the inner helix of the pore domain. Characterization of NavSulP and C-terminal deletion mutants NavSulP was cloned from S. pontiacus . The primary sequence of NavSulP has high identity (35.7%) and similarity (45.7%) with that of NaChBac, which was the first cloned NavBac from Bacillus halodurans [4] ( Fig. 1a ; Supplementary Fig. S1a ). NavSulP had a typical inward current ( Fig. 1b ). The half-maximum potentials for activation and inactivation of NavSulP were −31.2±1.9 mV ( n =9) and −62.1±1.0 mV ( n =6), respectively ( Supplementary Fig. S1b ). 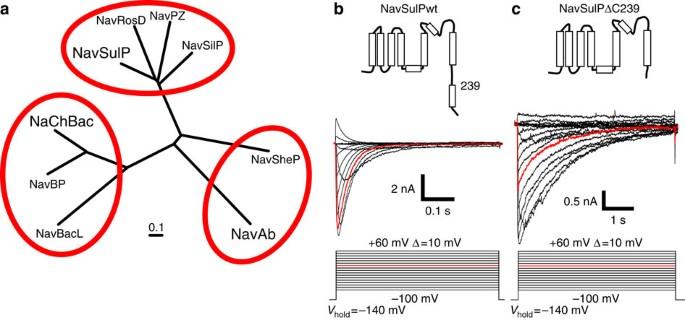Figure 1: Functional expression of wild-type and ΔC239 mutant channels of NavSulP. (a) Phylogenetic tree of the NavBacs, whose channel activities are confirmed. The three red circles indicate the cluster related to the primary sequence similarity. The branch lengths are proportional to the sequence divergence, with the scale bar corresponding to 0.1 substitutions per amino-acid site. (b) and (c) Schematic secondary structure and representative current traces of wild-type NavSulP and C-terminal deletion NavSulP (NavSulP ΔC239) resulting from the voltage protocol shown below, respectively. The current traces and voltage protocols drawn in red indicate those obtained at 0-mV membrane potential. The time constants of activation ( τ act ) and inactivation ( τ inact ) of NavSulP at 0 mV membrane potential were 2.76±0.45 ms and 40.6±7.0 ms ( n =8), respectively (the τ inact values of all the mutants at 0 mV membrane potential are summarized in Table 1 ). Figure 1: Functional expression of wild-type and ΔC239 mutant channels of NavSulP. ( a ) Phylogenetic tree of the NavBacs, whose channel activities are confirmed. The three red circles indicate the cluster related to the primary sequence similarity. The branch lengths are proportional to the sequence divergence, with the scale bar corresponding to 0.1 substitutions per amino-acid site. ( b ) and ( c ) Schematic secondary structure and representative current traces of wild-type NavSulP and C-terminal deletion NavSulP (NavSulP ΔC239) resulting from the voltage protocol shown below, respectively. The current traces and voltage protocols drawn in red indicate those obtained at 0-mV membrane potential. Full size image Table 1 Summary of the inactivation time constants. Full size table The C-terminal deletion of NavSulP (NavSulPΔC239) dramatically reduced (~40-fold) the inactivation rate at 0 mV membrane potential ( τ inact =1,701±421 ms: n =4), whereas the activation rate ( τ act =7.96±0.3 ms: n =4) was a little slower than that of wild-type channels ( Fig. 1c ). Two other deletion mutants (ΔC250 and ΔC257) also had slower inactivation rates ( Supplementary Fig. S2 ). The inactivation rates of the three deletion mutants were consistently slower than those of wild-type channels at various membrane potentials ( Fig. 2a; Table 1 ). The voltage producing the maximum current in the deletion mutants was ~10–~20 mV lower than that in wild-type NavSulP ( Fig. 2b–e ). The half-maximum potentials ( V 1/2 ) for inactivation of the three mutants were also lower (~15–~25 mV) than that of wild-type NavSulP ( Fig. 2f ; the values of V 1/2 for inactivation of all the mutants are summarized in Supplementary Table S1 ). The C-terminal deletion of NavSulP caused the negative shift of the voltage-dependence of channel gating as well as the reduction of the inactivation rate. 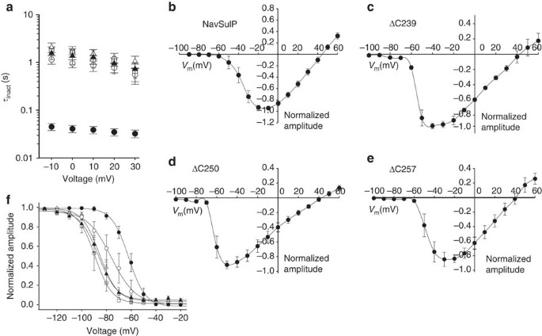Figure 2: Inactivation time constants and voltage-dependence of NavSulP and C-terminal deletion mutants. (a) The inactivation time constants (τinact) of NavSulP wild type (closed circle,n=8), ΔC239 (open triangle,n=4), ΔC250 (open square,n=4), ΔC257 (open circle,n=6) and tandemΔC239 (closed triangle,n=5) measured from the current traces elicited by step pulses from holding potential at −140 mV. The value ofτinactwas defined as the time from the peak current to 1/eof the peak current. (b–e) Mean peak current-voltage (I/V) relation of NavSulP wild type (n=8), ΔC239 (n=4), ΔC250 (n=4) and ΔC257 (n=6), normalized by the maximum current, respectively. (f) Steady-state inactivation curves for NavSulP wild type (n=6), ΔC239 (n=6), ΔC250 (n=4), ΔC257 (n=6) and tandemΔC239 (n=5). After a 2-second prepulse (from −120 to −20 mV, increments of +10 mV), the wild-type channel was inactivated to a steady-state level and reactivated by a second depolarization pulse (+20 mV). For the C-terminal deletion mutants, a 15-second prepulse (from −130 to −20 mV, increments of +10 mV) was used. All values are presented as mean±standard error. Figure 2: Inactivation time constants and voltage-dependence of NavSulP and C-terminal deletion mutants. ( a ) The inactivation time constants ( τ inact ) of NavSulP wild type (closed circle, n =8), ΔC239 (open triangle, n =4), ΔC250 (open square, n =4), ΔC257 (open circle, n =6) and tandemΔC239 (closed triangle, n =5) measured from the current traces elicited by step pulses from holding potential at −140 mV. The value of τ inact was defined as the time from the peak current to 1/ e of the peak current. ( b – e ) Mean peak current-voltage ( I / V ) relation of NavSulP wild type ( n =8), ΔC239 ( n =4), ΔC250 ( n =4) and ΔC257 ( n =6), normalized by the maximum current, respectively. ( f ) Steady-state inactivation curves for NavSulP wild type ( n =6), ΔC239 ( n =6), ΔC250 ( n =4), ΔC257 ( n =6) and tandemΔC239 ( n =5). After a 2-second prepulse (from −120 to −20 mV, increments of +10 mV), the wild-type channel was inactivated to a steady-state level and reactivated by a second depolarization pulse (+20 mV). For the C-terminal deletion mutants, a 15-second prepulse (from −130 to −20 mV, increments of +10 mV) was used. All values are presented as mean±standard error. Full size image In contrast to NavSulP, the inactivation rate is not altered in a NaChBac C-terminal deletion mutant [14] . Phylogenetic analysis of previously cloned NavBacs showed that they can be divided into three clusters ( Fig. 1a ). We measured the C-terminal deletion mutants of two other NavBacs (NavBacL and NavSheP) [7] , belonging to a different cluster than NavSulP. NavBacLΔC246 and NavShePΔC245 showed slightly slower inactivation rates than the wild-type channels ( Supplementary Fig. S3 ). The voltage inducing the maximum current and V 1/2 for channel inactivation, was similar to that of wild-type channels ( Supplementary Table S1 ). The crystal structure of NaK–NavSulPC239 chimera channel To understand the structural and functional role of the C-terminal region of NavSulP in the inactivation, the crystal structure of the C-terminal region of NavSulP was determined in a NaK–NavSulP chimera channel at 3.2 Å resolution, because the full-length NavSulP crystal was not available. The NaK channel is a tetrameric cation channel whose structure was determined at high resolution [15] , [16] . The C-terminal region from Thr239 of NavSulP (NavSulPC239) was grafted to the C-terminal Glu114 of a full-length NaK channel ( Supplementary Fig. S4 ). The chimera channel was well purified and crystallized. The structure of the chimera channel was determined by molecular replacement using the structure of a full-length NaK channel (pdb code: 2AHY (ref. 15 )) as the initial model. Data collectiyon and refinement statistics are summarized in Table 2 . Table 2 Data collection and refinement statistics. Full size table The structure of the NaK–NavSulPC239 chimera channel revealed that the transmembrane pore domain of the chimera channel formed a closed channel, like that of non-chimeric full-length NaK channels, and the C-terminal region of NavSulP was a well-ordered, 4HB structure extending away from the membrane ( Fig. 3a ). The asymmetric unit in the crystal lattice contained two monomers. The tetrameric channel had a two-fold symmetry rather than a four-fold symmetry. On the basis of the sequence similarity among previously cloned NavBacs ( Supplementary Fig. S1a ), the C-terminal 4HB is a common structure in NavBacs. 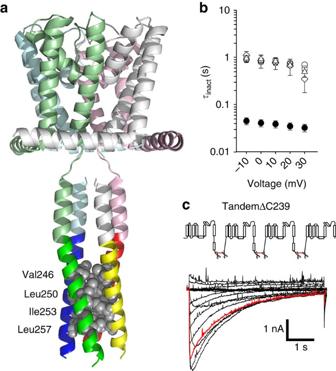Figure 3: Crystal structure of full-length NaK–NavSulP C239 chimera channel. (a) Crystal structure of the chimera channel of the full-length NaK and NavSulP C239. The C-terminal region of NavSulP forms a four-helix bundle (4HB). Each α-helix of the NavSulP subunit is represented in green, yellow, red and blue. The NaK channel is coloured by light green, white, pink and light cyan, corresponding to each NavSulP subunit. The side chains of hydrophobic residues that compose the hydrophobic core of the 4HB are shown as grey space-filling models. The location of Val246, Leu250, Ile253 and Leu257 is shown at the left side of the 4HB. (b) The inactivation time constants of V246R, L250R, I253R and L257R mutants of NavSulP, measured from the current traces elicited by step pulses from holding potential at −140 mV. The time constant of NavSulP wild type (closed circle,n=8), V246R (open circle,n=4), L250R (open square,n=4), I253R (open diamond,n=4) and L257R (open triangle,n=5) are represented as mean±standard error. (c) Schematic secondary structure and representative current traces of tandem-repeated NavSulPΔC239, resulting from same voltage protocol as that of the C-terminal deletion mutants. Four copies of NavSulP were connected by 28 amino acid-long linkers, which are indicated by the red lines. Thrombin recognition sites are indicated by the scissors. Tandem-repeated NavSulPΔC239 is composed of three wild-type NavSulP and one NavSulPΔC239 of the fourth repeat. The current trace drawn in red was obtained at 0-mV voltage. Figure 3: Crystal structure of full-length NaK–NavSulP C239 chimera channel. ( a ) Crystal structure of the chimera channel of the full-length NaK and NavSulP C239. The C-terminal region of NavSulP forms a four-helix bundle (4HB). Each α-helix of the NavSulP subunit is represented in green, yellow, red and blue. The NaK channel is coloured by light green, white, pink and light cyan, corresponding to each NavSulP subunit. The side chains of hydrophobic residues that compose the hydrophobic core of the 4HB are shown as grey space-filling models. The location of Val246, Leu250, Ile253 and Leu257 is shown at the left side of the 4HB. ( b ) The inactivation time constants of V246R, L250R, I253R and L257R mutants of NavSulP, measured from the current traces elicited by step pulses from holding potential at −140 mV. The time constant of NavSulP wild type (closed circle, n =8), V246R (open circle, n =4), L250R (open square, n =4), I253R (open diamond, n =4) and L257R (open triangle, n =5) are represented as mean±standard error. ( c ) Schematic secondary structure and representative current traces of tandem-repeated NavSulPΔC239, resulting from same voltage protocol as that of the C-terminal deletion mutants. Four copies of NavSulP were connected by 28 amino acid-long linkers, which are indicated by the red lines. Thrombin recognition sites are indicated by the scissors. Tandem-repeated NavSulPΔC239 is composed of three wild-type NavSulP and one NavSulPΔC239 of the fourth repeat. The current trace drawn in red was obtained at 0-mV voltage. Full size image The amino-terminal region and transmembrane domain, derived from the NaK channel up to Leu 98, was almost the same as that of the full-length NaK channel (averaged root-mean-square deviation=0.65 Å). The cytosolic part of the inner helix, comprising residues from Asn101 to Gln103, of the chimera channel formed an extended loop ( Supplementary Fig. S5a,b ), although the inner helix of the non-chimeric NaK channel formed an α-helix up to the C-terminus ( Supplementary Fig. S5c ). In the NaK channel structure (pdb code: 3E86 (ref. 16 )), the Pro105 imino group formed hydrogen bonds with the carbonyl group of Val100, instead of Asn101 ( Supplementary Fig. S5c ). Isolation of Asn101 from the hydrogen-bond networks would make the α-helix turn before Pro105 intrinsically unstable and flexible. In the structure of the chimera channel, the carbonyl groups of Val100 and Asn101 did not form hydrogen bonds with the Pro105 imino group, which might extend the α-helix ( Supplementary Fig. S5b ). This structural flexibility could absorb the artificial contortion of the graft of the NavSulP C-terminal region. The residues from Leu104 to Glu114, which derive from the C-terminus of the NaK channel, also participated in the 4HB, but no interaction was observed in the part of the 4HB derived from the NaK channel. The hydrophobic core of the 4HB The structure suggests that the main interaction of the 4HB formation is a hydrophobic interaction among Val246, Leu250, Ile253 and Leu257 ( Fig. 3a ). All 4 single-point mutations affecting the hydrophobic core (V246R, L250R, I253R and L257R) reduced the inactivation rates ( Fig. 3b ; Table 1 ). The voltage-dependence of their inactivation and the voltage inducing maximum current were negatively shifted compared with those of the wild-type channel ( Supplementary Table S1 ; Supplementary Fig. S6 ), and were similar to those of the C-terminal deletion mutants. These 4 residues from each subunit (16 hydrophobic residues) comprise the tightly packed hydrophobic core on the axis at the centre of the pore domain. The inactivation rate and voltage dependency of the mutant channel of NavSulP lacking one of four C-terminal helices, which is a covalently linked tandem tetramer in which the fourth subdomain lacks the C-terminal region (TandemΔC239), were similar to that of the C-terminal deletion mutant ( Figs 2 and 3c ; Supplementary Fig. S6e ). Four helices from each of the four channel subunits were required for fast inactivation, as in the wild type. These findings suggest that the weaker interactions or breakdown of the 4HB reduce the inactivation rate. The other intersubunit interactions of the 4HB The C-terminal 4HB of NavSulP had two other intersubunit interactions ( Fig. 4 ). Arg243 formed a hydrogen bond with Thr239 of the adjacent helix and interacted with Tyr242 by CH/ π stacking ( Fig. 4a ). Accordingly, the inactivation rate and voltage dependency of NavSulP R243E were similar to that of the C-terminal deletion mutant ( Fig. 4c ; Supplementary Fig. S7 ). Neutral mutations of Arg243 and Thr239 (R243A and T239V) also reduced the inactivation rate ( Fig. 4c ). The Y242A mutations reduced the inactivation rate, whereas the inactivation rate of NavSulP Y242F was not significantly different from that of the wild-type protein ( Fig. 4c ). These findings suggest that the interactions of Arg243, the hydrogen bond with Thr239, and the CH/π stacking with Tyr242, support the formation of the 4HB and accelerate the inactivation rate. 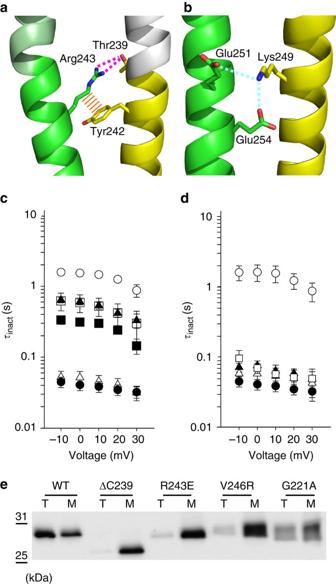Figure 4: The intersubunit interaction of the 4HB. (a) Intersubunit interaction around Arg243. Hydrogen bond and CH/πstacking are indicated by dashed magenta and orange lines, respectively. (b) The ion bridge interaction of Lys249. Dashed cyan line represents ion bridges. (c,d) Mutational effect of the residues that participated in the interaction of Arg243 (c) and Lys249 (d) for the inactivation time constants. The inactivation time constants were measured from the current traces elicited by step pulses from holding potential at −140 mV. The time constant of NavSulP wild type (closed circle,n=8), R243E (open circle,n=4), Y242A (closed triangle,n=6), Y242F (open triangle,n=5), T239V (closed square,n=5) and R243A (open square,n=4) are represented in (c). The time constant of NavSulP wild type (closed circle,n=8), K249E (open circle,n=5), E251K (closed triangle,n=4), E254K (open triangle,n=4) and E251K/E254K (open square,n=4), are represented in (d). All values are presented as mean±standard error. (e) Sodium dodecyl sulphate-polyacrylamide gel electrophoresis analysis of tetramer and monomer fractions of NavSulP wild-type (WT) and mutants in size-exclusion chromatography. T and M indicate the tetramer and monomer fractions of NavSulP proteins in size-exclusion chromatography, respectively. To evaluate the amount of protein, proteins were denatured to monomers by sodium dodecyl sulphate treatment. The band intensities of the T and M lanes represent the amount of tetrameric channels and dissociated monomers, respectively. Most NavSulPΔC239 were dissociated to monomers and unable to form channel tetramers. Figure 4: The intersubunit interaction of the 4HB. ( a ) Intersubunit interaction around Arg243. Hydrogen bond and CH/ π stacking are indicated by dashed magenta and orange lines, respectively. ( b ) The ion bridge interaction of Lys249. Dashed cyan line represents ion bridges. ( c , d ) Mutational effect of the residues that participated in the interaction of Arg243 ( c ) and Lys249 ( d ) for the inactivation time constants. The inactivation time constants were measured from the current traces elicited by step pulses from holding potential at −140 mV. The time constant of NavSulP wild type (closed circle, n =8), R243E (open circle, n =4), Y242A (closed triangle, n =6), Y242F (open triangle, n =5), T239V (closed square, n =5) and R243A (open square, n =4) are represented in ( c ). The time constant of NavSulP wild type (closed circle, n =8), K249E (open circle, n =5), E251K (closed triangle, n =4), E254K (open triangle, n =4) and E251K/E254K (open square, n =4), are represented in ( d ). All values are presented as mean±standard error. ( e ) Sodium dodecyl sulphate-polyacrylamide gel electrophoresis analysis of tetramer and monomer fractions of NavSulP wild-type (WT) and mutants in size-exclusion chromatography. T and M indicate the tetramer and monomer fractions of NavSulP proteins in size-exclusion chromatography, respectively. To evaluate the amount of protein, proteins were denatured to monomers by sodium dodecyl sulphate treatment. The band intensities of the T and M lanes represent the amount of tetrameric channels and dissociated monomers, respectively. Most NavSulPΔC239 were dissociated to monomers and unable to form channel tetramers. Full size image Another interaction was the salt-bridge of Lys249 with Glu251 and Glu254 of adjacent subunits ( Fig. 4b ). This type of interaction was not observed in other helical pairs in the asymmetric unit of the crystal lattice. The inactivation rate of NavSulP K249E was similar to that of NavSulPΔC239 ( Fig. 4d ). The E251K and/or E254K mutations, however, did not significantly reduce the inactivation rate ( Fig. 4d ). These results suggest that Lys249 is involved in the interaction with residues other than Glu251 and Glu254 for accelerating channel inactivation. The role of the 4HB in stabilization of channel tetramer In addition to accelerating inactivation, NavSulP 4HB promotes the formation of the channel tetramer. Purified wild-type protein of NavSulP, migrated as two distinct peaks in size-exclusion chromatography, and crosslinkage analysis with glutaraldehyde indicated that the larger molecular weight peak comprised a NavSulP tetramer, and the other peak comprised a dissociated NavSulP monomer ( Supplementary Fig. S8a,b ). Most of the NavSulPΔC239 migrated as monomers ( Fig. 4e ; Supplementary Fig. S8c ). The R243E and V246R mutations also increased the number of monomer peaks ( Fig. 4e ; Supplementary Fig. S8d,e ). These mutations destabilized the tetramer formation of the channels in addition to reducing their inactivation rate. The 4HB accelerates the inactivation via the inner helix The 4HB formation is thought to modify the inactivation mechanism of the pore domain, because the C-terminal deletion mutants were functional and capable of full inactivation, albeit at a slower rate ( Fig. 1c ). We previously demonstrated that mutation of the conserved glycine residue of the cytosolic part of the inner helix to alanine reduced the NavBacs inactivation rate [7] . The 4HB was directly connected to the inner helix ( Supplementary Fig. S1a ), and superimposition of the structure of the chimera channel and NavAb (pdb code: 3RVY [8] ) ( Fig. 5a ) showed that Gly221 of NavSulP, which corresponds to the conserved glycine of the inner helix, located in the connection between the inner helix and the 4HB (blue in Fig. 5b ). NavSulP G221A also showed a slower inactivation rate ( τ inact =1850±368 ms at 0 mV membrane potential: n =6) than any other deletion or point mutation ( Fig. 5c ), but the purified protein of NavSulP G221A had a tetrameric channel that was similar to the wild-type channel in size-exclusion chromatography ( Fig. 4e ; Supplementary Fig. S8f ). Moreover, the C-terminal deletion mutant of NavSulP G221A (NavSulP G221AΔC239) showed an extremely slow inactivation rate ( τ inact =5088±1143 ms at 0 mV membrane potential: n =5) and generated a large deactivation tail current after 90-second depolarization ( Fig. 5d ), which indicated that stabilization of the inner helix partially defeated the inactivation mechanism of the pore domain. Therefore, the inner helix is suggested to be involved in the inactivation mechanism of the pore domain, and the formation of the 4HB would modify the inactivation mechanism through the inner helix. 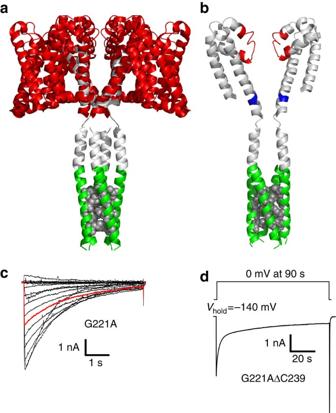Figure 5: Comparison of the structure of the chimera channel of NaK–NavSulP C239 with that of NavAb. (a) Superimposition of the inner helix and the C-terminal 4HB of the NaK–NavSulPC239 chimera channel structure and whole NavAb structure (PDB code, 3RVZ) by ribbon diagrams. The inner helices of the chimera channel are superimposed on those of NavAb. The NaK part of the chimera channel is shown in white, and the NavSulP part of the chimera channel is shown in green. The NavAb is shown in red. The side-chains of the residues of the hydrophobic core are indicated by grey-coloured ball models (Val246, Leu250, Ile253 and Leu257 are in grey). (b) The ribbon diagram of the pore domain of NavAb and the superimposed 4HB of the chimera channel. The part of the selectivity filter and the residues participating in the intersubunit hydrogen-bond network around the selectivity filter is indicated in red, and the residue corresponding to the conserved glycine in the inner helix is in blue. (c) Representative traces of the current of NavSulP G221A resulting from same voltage protocol as that of the C-terminal deletion mutants. The current trace drawn in red was obtained at 0-mV voltage. (d) Representative trace of the current of NavSulP G221A ΔC239 resulting from the 0-mV voltage depolarization protocol (90 s) shown above. Figure 5: Comparison of the structure of the chimera channel of NaK–NavSulP C239 with that of NavAb. ( a ) Superimposition of the inner helix and the C-terminal 4HB of the NaK–NavSulPC239 chimera channel structure and whole NavAb structure (PDB code, 3RVZ) by ribbon diagrams. The inner helices of the chimera channel are superimposed on those of NavAb. The NaK part of the chimera channel is shown in white, and the NavSulP part of the chimera channel is shown in green. The NavAb is shown in red. The side-chains of the residues of the hydrophobic core are indicated by grey-coloured ball models (Val246, Leu250, Ile253 and Leu257 are in grey). ( b ) The ribbon diagram of the pore domain of NavAb and the superimposed 4HB of the chimera channel. The part of the selectivity filter and the residues participating in the intersubunit hydrogen-bond network around the selectivity filter is indicated in red, and the residue corresponding to the conserved glycine in the inner helix is in blue. ( c ) Representative traces of the current of NavSulP G221A resulting from same voltage protocol as that of the C-terminal deletion mutants. The current trace drawn in red was obtained at 0-mV voltage. ( d ) Representative trace of the current of NavSulP G221A ΔC239 resulting from the 0-mV voltage depolarization protocol (90 s) shown above. Full size image The C-terminal region of NavSulP has a novel mechanism for accelerating the channel inactivation rate. The inactivation of NavBacs is thought to only occur through the C-type inactivation mechanism because NavBacs lack an obvious cytoplasmic domain required for inactivation, such as an 'inactivation peptide' [17] or an 'IMF motif' [18] . The C-type inactivation mechanism of the sodium channel remains unclear, while that of the potassium channel is well understood based on the structure of KcsA. In the case of KcsA, it is thought that a large rotation of the activation gate, which is the cytosolic part of the inner helix, causes the collapse of the selectivity filter during C-type inactivation [19] , [20] . The 4HB of KcsA reduces the C-type inactivation rate by restricting the activation-gate rotation with the formation of the 4HB [21] , [22] . The NavSulP 4HB contained a hydrophobic interaction similar to that of KcsA. Furthermore, the NavSulP 4HB also seems to restrict the movement of the inner helix, because the 4HB-grafted NaK–NavSulPC239 chimera channel does not change the closed structure of the original NaK channel (pdb accession code: 2AHY (ref. 15 )). Although they have similar roles in the restriction of the cytosolic part of the inner helix, the 4HB of NavSulP and KcsA have opposite effects on the inactivation rate. The findings of this study suggest that the scheme of NavSulP inactivation differs from that of KcsA C-type inactivation. The structure of NavAb [8] allows us to evaluate the effect of the 4HB formation on the inner helix of the NavSulP pore domain. The pore domain of NavAb seems to form a closed structure, although the voltage sensor domains are in an activated state [8] . The cytosolic C-terminal region of NavAb was not determined, but located in the crystal lattice. On the basis of the sequence similarity, the C-terminal region of NavAb would form the 4HB and make the inner helix a closed form, as does that of KcsA and NavSulP. On depolarization, while the voltage sensor domains open the activation gate, 4HB would generate a counter force to close the gate of the inner helix. The counter force could promote the conformational change of the inner helix to inactivate the pore domain ( Fig. 6 ). Stabilization of the inner helix with the G221A mutation reduced the inactivation rate ( Fig. 5c ). Formation of the 4HB would require more time to promote the conformational change of the rigid inner helix of NavSulP G221A than that of wild-type NavSulP ( Supplementary Fig. S9a ). The inner helix of C-terminal deletion NavSulP would be free from the counter force of 4HB formation, and spontaneously enter into the inactivated state with a slower rate ( Supplementary Fig. S9b ). This could be the reason for the slower inactivation rate of the C-terminal deletion mutant of NavSulP. 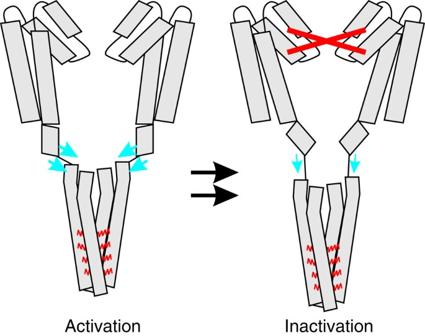Figure 6: Hypothetical model of the role of the NavSulP 4HB formation in inactivation. The front and rear subunits of the transmembrane part were removed for clarity. The hinge of the inner helix indicates the position of Gly221. The red lines in 4HB indicate the interaction of the hydrophobic core. The blue arrows indicate the tension of the 4HB formation on the inner helix. The double black arrows indicate the accelerated transition from the open state to the inactivated state by formation of the 4HB. Figure 6: Hypothetical model of the role of the NavSulP 4HB formation in inactivation. The front and rear subunits of the transmembrane part were removed for clarity. The hinge of the inner helix indicates the position of Gly221. The red lines in 4HB indicate the interaction of the hydrophobic core. The blue arrows indicate the tension of the 4HB formation on the inner helix. The double black arrows indicate the accelerated transition from the open state to the inactivated state by formation of the 4HB. Full size image It is possible that the inactivation of NavBacs only occurs through the collapse of the selectivity filter, which is called 'C-type inactivation', because the inactivation of NaChBac is very sensitive to mutations around the selectivity filter [23] , [24] . The selectivity filter of NavAb (red in Fig. 5b ) is elaborately constructed with a well-developed intersubunit hydrogen-bond network [8] . Similar hydrogen-bond networks are not observed in the selectivity filter of the potassium channel [25] , [26] . If the selectivity filter breaks down in the inactivation of NavSulP, the 4HB might promote the collapse of the delicate selectivity filter through the conformational change of the inner helix. The structure of NavAb, however, was the only structure in the pore domain of Nav. To reveal the inactivation mechanism of NavBacs, it is necessary to determine the structure of the pore domain of NavSulP and homologues in other states and perform a detailed comparison of them. The formation of NavSulP 4HB had another effect on channel activity in addition to accelerating the channel inactivation rate. The deletion and destabilization of 4HB caused a negative shift of the voltage producing the maximum current and steady-state inactivation as well as reduction of the inactivation rate ( Supplementary Table 1 and the current-voltage relation curves of Fig. 2 ; Supplementary Figs S6 and S7 ). The negative shift of the voltage producing the maximum current indicated that these mutants could enter open state more easily at negative membrane potentials. NavBacs are spontaneously inactivated after activation. Therefore, the negative shift of the steady-state inactivation of the 4HB disrupted mutants was thought to be caused by the negative shift of activation. This result suggested that the formation of the cytosolic 4HB would have a supportive role for closing the activation gate of the inner helix in the resting state, whereas the voltage sensor domain could be the main player for keeping the pore domain closed. As well as the acceleration of inactivation rate could reduce excess ion flux after activation, the 4HB formation could contribute to suppress accidental ion flux even in the resting state. The 4HB of NavSulP has a remarkable role in the stabilization of the channel tetramer as well as the modulation of channel properties, but those of the other homologues (NaChBac [14] , NavBacL and NavSheP) had a smaller impact on the inactivation rate ( Supplementary Fig. S3 , Supplementary Table S1 ). The length of the loop between the inner helix and the C-terminal 4HB varies for each NavBacs homologue. The primary sequence alignment showed that members of the NavSulP group have a shorter loop than those of the other groups ( Fig. 1a ; Supplementary Fig. S1a ). Furthermore, the residues of NavSulP (Thr239, Tyr242 and Arg243), which are involved in the intersubunit interactions of the 4HB, are only conserved in the NavSulP group. Acceleration of the inactivation rate by the 4HB formation might be a unique mechanism of NavSulP and channels in the same cluster. Although the C-terminal deletion of the NavBacs of Bacillus species (NaChBac and NavBacL) did not affect the inactivation rate, our previous study showed that stabilization of the inner helix by a glycine-to-alanine mutation also reduced their inactivation rate [7] . In the Bacillus species cluster, the mobility of the inner helix, which is not modulated by the formation of the 4HB, would regulate their inactivation rate as well as that of NavSulP. NavSheP and NavAb have no glycine residue in the inner helix [7] , [8] , and their inactivation rate would be less modulated by the 4HB. The inactivation rates of NavBacs are thought to be regulated by the rigidity of the inner helix and the effect of the cytosolic 4HB in a homologue-dependent manner. NavSulP seems to depend on the cytosolic C-terminal region to modulate the channel activity more than the other homologues. Tetramerization of the cytosolic C-terminal helices is observed in the crystal structure of various tetrameric ion channels, and is thought to have various roles in channel function [9] , [21] , [27] . The NavSulP 4HB has a unique role in stabilization of the channel tetramer as well as in acceleration of the inactivation rate. Formation of the 4HB accelerates the inactivation rate of NavSulP, but reduces that of KcsA. Our results suggest that the scheme of the inactivation of sodium channels is different from that of potassium channels. Cloning of NavSulP and site-directed mutagenesis The NavSulP DNA was cloned from S. pontiacus (JCM No. 21789), as described previously [7] . The following primers were used for cloning: 5′-CGCGGATCCATGGTGGGCACGGTAAACATG-3′ and 5′-CGCGGATCCCTGTCGGCTGTGCTCTGCCAG-3′. Site-directed mutagenesis was accomplished by polymerase chain reaction, using high-fidelity Pfu DNA polymerase (method by Stratagene). To generate the series of tandem NavSulP tetramers, four copies were covalently connected by LVPRGSXXGSSHHHHHHSSGLVPRGSSH linkers, in which 'XX' denotes the amino acids resulting from the translation of the recognition sites for the restriction enzymes (EP, TR and GT for the Eco RI, Mlu I and Acc 65I recognition sites, respectively). All clones were confirmed by DNA sequencing. Expression and purification of NavSulP Proteins were expressed in the Escherichia coli KRX strain (Promega). Cells were grown at 37 °C to an OD 600 of 0.8, induced with 0.1% rhamnose (Wako), and grown for 16 h at 18 °C. The cells were suspended in TBS buffer (20 mM Tris–HCl pH 8.0, 150 mM NaCl), and lysed using a French Press (SLM AMINCO) at 12,000 psi. Membranes were collected by centrifugation (100,000 g , 1 h, 4 °C) and solubilized by homogenization in TBS buffer containing 40 mM CYMAL-6 (Anatrace). After centrifugation (40,000 g , 30 min, 4 °C), the supernatant was loaded onto a HIS-Select cobalt affinity gel column (Sigma). The column was washed with 10 mM imidazole in TBS buffer containing 3 mM CYMAL-6 and 0.1 mg ml −1 E. coli polar lipid (Avanti), and the protein was eluted with 300 mM imidazole. Eluted protein was purified on a Superdex-200 gel filtration column in 150 mM NaCl, 20 mM HEPES-NaOH pH 8.0, 3 mM CYMAL-6 and 0.1 mg ml −1 E. coli polar lipid. The crosslinking reaction with 1.0 mM glutaraldehyde was performed for 30 min at 37 °C. Purified proteins were resolved on 7.5–20% sodium dodecyl sulphate-polyacrylamide gel electrophoresis gradient gels (Wako) and stained with silver staining. Electrophysiology of mammalian cells All electrophysiological experiments were performed as described previously [7] . The pipette solution contained 105 mM CsF, 35 mM NaCl, 10 mM EGTA and 10 mM HEPES-CsOH pH 7.4. The bath solution contained 150 mM NaCl, 1.5 mM CaCl 2 , 1 mM MgCl 2 , 2 mM KCl, 10 mM HEPES-NaOH pH 7.4 and 10 mM glucose. Whole-cell currents were recorded with a patch–clamp amplifier (EPC10). Patch electrodes were pulled from borosilicate glass and had resistances of 1–3 MΩ. Current amplitudes ranged from 500 pA to 10 nA. Series resistance was compensated up to 70% to reduce all series resistance errors to <20 mV. Cells in which series resistance was >10 MΩ were discarded. For measurement of tandem-repeated tetramers, 10 U ml −1 thrombin was added to the pipette solution. All experiments were conducted at 25±2 °C. The activation time constant ( τ act ) was defined as the time from 10% to 90% of the peak current. The inactivation time constant ( τ inact ) was defined as the time from the peak current to 1/ e of the peak current. All results are presented as mean±standard error. Purification of the NaK–NavSulP chimera channel The NaK channel from Bacillus weihenstephanensis (NBRC No. 101238) was cloned into the modified pET-21b vector. The NaK–NavSulP chimera channel was constructed by inserting the C-terminal region of NavSulP (239–263) between the C-terminal end of NaK and the thrombin digestion site of pET-21b vector. The chimera channel was expressed in E. coli KRX cultures at 25 °C. The purification procedure of the chimera channel was similar to that of full-length Nav homologues. In this procedure, CYMAL-6 was replaced with DM (n-decyl-β-d-maltopyranoside, Anatrace, anagrade), and E. coli polar lipid was removed. For membrane solubilization, 20 mM DM was used. In the wash and eluate, 5 mM DM was used. Eluate of the chimera channel was concentrated for further purification. Concentrated protein (~15 mg ml −1 ) was purified on a Superdex-200 gel filtration column in 150 mM NaCl, 20 mM Tris–HCl pH 7.5, 5 mM DM. Structure determination of the chimera channel Crystals were grown by hanging-drop vapour diffusion at 20 °C by mixing 2-μl volumes of protein solution (4–6 mg ml −1 ) and reservoir solution (19–21% polyethylene glycol monomethyl ether 550, 50 mM magnesium nitrate and 100 mM sodium citrate, pH 5.6). All data were collected at BL38B1 (Wavelength: 0.978 Å) of SPring-8 and processed using HKL2000 (ref. 28 ). The crystals were of space group P 3 1 21 with cell dimensions a = b =104.3, c =104.8, α=β=90°, γ=120° and contained two subunits per asymmetric unit. The four-fold axis of the channel tetramer coincided with one of the crystallographic two-fold symmetry axes. The initial phase was obtained by the molecular replacement method with PHASER [29] using the full-length NaK channel (pdb code: 2AHY [15] ) as the initial model at 3.8 Å. The model was constructed in COOT [30] and refined in refmac5 (ref. 31 ) to 3.2 Å with R work 29.4% and R free 32.0%. Acccession codes: The DNA sequence of NavSulP and NaK channel has been deposited in the DNA Data Bank of Japan under accession codes, AB617621 and AB617622 , respectively. Coordinates and structure factors for the NaK–NavSulP chimera channel have been deposited in the Protein Data Bank under accession code 3VOU . How to cite this article: Irie, K. et al . The C-terminal helical bundle of the tetrameric prokaryotic sodium channel accelerates the inactivation rate. Nat. Commun. 3:793 doi: 10.1038/ncomms1797 (2012).